Lck tyrosine kinase mediates β1-integrin signalling to regulate Schwann cell migration and myelination The interaction between laminin and β1-integrin on the surface of Schwann cells regulates Schwann cell proliferation, maturation and differentiation. However, the signalling mediators that fine-tune these outcomes are not fully elucidated. Here we show that lymphoid cell kinase is the crucial effector of β1-integrin signalling in Schwann cells. Lymphoid cell kinase is activated after laminin treatment of Schwann cells, while downregulation of β1-integrin with short interfering RNAs inhibits lymphoid cell kinase phosphorylation. Treatment of Schwann cells with a selective lymphoid cell kinase inhibitor reveals a pathway that involves paxillin and CrkII, which ultimately elevates Rac-GTP levels to induce radial lamellipodia formation. Inhibition of lymphoid cell kinase in Schwann cell-dorsal root ganglion cocultures and dorsal root ganglions from Lck −/− mice show a reduction of Schwann cell longitudinal migration, reduced myelin formation and internode length. Finally, Lck −/− mice exhibit delays in myelination, thinner myelin with abnormal g-ratios and aberrant myelin outfoldings. Our data implicate lymphoid cell kinase as a major regulator of cytoskeletal dynamics, migration and myelination in the peripheral nervous system. During embryonic development, Schwann cell (SC) progenitors arise from the neural crest and populate the spinal roots by proliferating and migrating along the extending axons. Immature SCs then wrap around large bundles of axons and initiate radial sorting, the process by which SCs recognize and segregate large calibre axons to establish a 1:1 relationship before myelination [1] . After sorting of the large calibre axons is complete, non-myelinating SCs form Remak bundles, which contain one SC and multiple small calibre axons separated by SC cytoplasm [2] . The primary extracellular signals that regulate and support SCs through development, axonal sorting and myelination are the neuregulin/ErbB axis (axonal) [3] , [4] , [5] , [6] and laminin/integrin (basal lamina) signalling [7] , [8] , [9] , [10] . In the mature peripheral nervous system (PNS), SCs are surrounded by a specialized basal lamina composed of a diverse group of extracellular matrix (ECM) proteins including collagen, proteoglycans and laminin, which provide a scaffold for cell adhesion and extracellular signalling critical for morphogenesis [11] , [12] . In SCs, laminin is the predominant ECM protein that regulates differentiation, and SC-specific loss of the γ1 subunit, found in all laminin isoforms, results in severe defects in axonal sorting, hypomyelination and inhibition of Remak bundle formation [13] , [14] , [15] . The cell surface receptors for laminins and other ECM proteins are integrins, a large family of heterodimeric receptors (αβ) of which SCs express α1β1, α6β1, α6β4 and α7β1 (ref. 16 ). Loss of β1-integrin in SCs results in severe hypomyelination due to defects in axonal radial sorting and radial lamellipodia formation [17] . Radial lamellipodia formation requires actin polymerization and cytoskeletal rearrangement that are in part regulated by Rho GTPases such as Cdc42 and Rac1, which act as molecular switches and are required for radial sorting of axons [18] , [19] , [20] . Rac1 is a downstream effector of β1-integrin regulation of axonal radial sorting, and overexpression of Rac1 can partially rescue the β1-integrin knockout (KO) hypomyelinating phenotype [21] . Rac1 mediates both axial extension of SC processes and radial lamellipodia formation, and it is hypothesized that an increased level of Rac1 is required for the switch from longitudinal elongation to radial lamellipodia formation [21] . However, the signal(s) that mediate the increased Rac1 levels following β1-integrin activation to induce radial lamellipodia formation have not been elucidated. In this study, we examined the role of lymphoid cell kinase (Lck), an Src kinase family member, as a mediator of β1-integrin signalling, which regulates cell migration, axonal sorting and myelination. Lck signalling through paxillin and CrkII regulates the levels of active Rac1 in SCs and mediates the dynamic formation of radial lamellipodia. Lck −/− SCs show reduced rate of migration on dorsal root ganglion (DRG) axons, and shorter and fewer internodes upon myelination. Furthermore, we show that Lck −/− mice exhibit a transient impairment of radial sorting of axons, delayed myelination, abnormal myelin thickness and the presence of aberrant myelin outfoldings. These results demonstrate that Lck is a crucial mediator of β1-integrin signalling in SCs and regulates SC cytoskeletal rearrangements, migration and the proper timing and integrity of myelination. β1-Integrin induces Lck phosphorylation in SCs Previously we have described a role of Lck in promoting proliferation in Mycobacterium leprae -infected human SCs through a non-canonical activation of Erk1/2 via PKCε (ref. 22 ). To determine whether a similar signalling pathway exists in non-infected SCs, we analysed Lck activity on β1-heregulin signalling and proliferation in rodent SCs. These studies showed that Lck is not an intermediate of neuregulin-ErbB3 signalling in SCs ( Supplementary Fig. S1 ). In addition, Lck does not appear to regulate SC proliferation, as no effects were seen in Lck −/− mouse SCs or during pharmacological inhibition of Lck in rat Schwann cells (RSCs) ( Supplementary Fig. S1 ). Next, we examined the effect of ECM signalling on Lck phosphorylation, as Src family members have a critical role in cell adhesion and migration [23] . In particular, Src family kinases (SFKs), Fyn and Lyn, mediate laminin/β1-integrin signalling during oligodendrocyte differentiation, and Src kinase acts downstream of laminin/β-dystroglycan signalling in SCs [24] , [25] , [26] . We treated serum- and growth factor-starved RSCs with mouse laminin (15 μg ml −1 ) and used an antibody generated specifically against phospho(Y394)-Lck ( Supplementary Fig. S2 and Methods). Significant endogenous Lck activation was observed in laminin-treated RSCs ( Fig. 1a , P <0.03). Similar activation of overexpressed Lck protein was detected in laminin-treated RSCs, which was significant at 10-min exposure ( Fig. 1b , P <0.008). Inhibition of β1-integrin expression by short interfering RNA (siRNA) inhibits the laminin-induced phosphorylation of Lck at the active site ( Fig. 1d ) without impeding RSC attachment to laminin-coated dishes (data not shown). Coexpression of siRNA (CTL or β1-integrin) and Lck plasmid for 48 h, followed by seeding RSCs on laminin-coated dishes, also induces phosphorylation of overexpressed Lck, which is reduced after inhibition of β1-integrin expression by siRNAs ( Fig. 1e ). 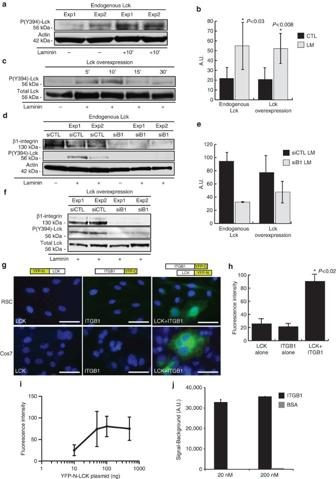Figure 1: Laminin-induced interaction of β1-integrin with Lck mediates Lck phosphorylation in SCs. (a,b) Active site (Y394) phosphorylation of endogenous Lck is induced after 10-min incubation with laminin (15 μg ml−1) in serum-starved SCs. Panel depicts representative western blot from two independent experiments. (b) Graph shows densitometric quantification of western blots for Lck phosphorylation from endogenous Lck (P<0.03,n=4) (a) and overexpressed Lck (P<0.008,n=5) (c), error bars represent ±s.d. (c) SCs overexpressing Lck were treated with 15 μg ml−1laminin, and lysates were analysed for Lck phosphorylation. Lck is transiently activated (5–10 min) in response to laminin treatment. Quantification of Lck phosphorylation is shown inb. (d–f) Phosphorylation of endogenous Lck (d) or overexpressed Lck (f) was reduced following downregulation of β1-integrin with a specific siRNA but not with a control non-targeting siRNA, and quantification of western blots is shown (e,n=2). (g)In vivointeraction between Lck and β1-integrin is identified by BiFC in SCs and Cos7 cells. BiFC constructs were generated by fusing Lck to YFP-N (a.a. 1–158) and β1-integrin to YFP-C (a.a. 159–235). Coexpression in both SCs and Cos7 cells showed YFP fluorescence at the cell membrane. Expression of either construct alone did not produce YFP fluorescence. Scale bars represent 50 μm. (h) Average fluorescence intensities of YFP constructs. Intensity values correspond to 3-s exposure with background removed. Expression of Lck-YFP-N or ITGB1-YFP-C alone represents cell autofluorescence. Cells below this intensity level were not analysed in the LCK+ITGB1 experiments. Average fluorescence intensity was significantly increased during coexpression of Lck-YFP-N and ITGB1-YFP-C in Cos7 cells (P<0.03 vs Lck alone and ITGB1 alone,n=2 independent experiments, error bars represent ±s.d.). (i) Cell fluorescence intensity correlates to increasing YFP-N-LCK expression in Cos7 cells (n=3 independent experiments,yaxis=log10, error bars represent ±s.d). (j) Active Lck binds directly to β1-integrin in a chemiluminescence binding assay using recombinant human proteins (Meso Scale Discovery). Representative signal measurements are shown for active Lck bound to β1-integrin, with saturating concentrations of active Lck and β1-integrin of 20 nM and 200 nM (n=duplicate wells, error bars represent ±s.d). Non-specific binding (BSA) showed a negligible signal. Statistical significance was determined by two-tailed Student’st-test. Figure 1: Laminin-induced interaction of β1-integrin with Lck mediates Lck phosphorylation in SCs. ( a , b ) Active site (Y394) phosphorylation of endogenous Lck is induced after 10-min incubation with laminin (15 μg ml −1 ) in serum-starved SCs. Panel depicts representative western blot from two independent experiments. ( b ) Graph shows densitometric quantification of western blots for Lck phosphorylation from endogenous Lck ( P <0.03, n= 4) ( a ) and overexpressed Lck ( P <0.008, n= 5) ( c ), error bars represent ±s.d. ( c ) SCs overexpressing Lck were treated with 15 μg ml −1 laminin, and lysates were analysed for Lck phosphorylation. Lck is transiently activated (5–10 min) in response to laminin treatment. Quantification of Lck phosphorylation is shown in b . ( d – f ) Phosphorylation of endogenous Lck ( d ) or overexpressed Lck ( f ) was reduced following downregulation of β1-integrin with a specific siRNA but not with a control non-targeting siRNA, and quantification of western blots is shown ( e , n= 2). ( g ) In vivo interaction between Lck and β1-integrin is identified by BiFC in SCs and Cos7 cells. BiFC constructs were generated by fusing Lck to YFP-N (a.a. 1–158) and β1-integrin to YFP-C (a.a. 159–235). Coexpression in both SCs and Cos7 cells showed YFP fluorescence at the cell membrane. Expression of either construct alone did not produce YFP fluorescence. Scale bars represent 50 μm. ( h ) Average fluorescence intensities of YFP constructs. Intensity values correspond to 3-s exposure with background removed. Expression of Lck-YFP-N or ITGB1-YFP-C alone represents cell autofluorescence. Cells below this intensity level were not analysed in the LCK+ITGB1 experiments. Average fluorescence intensity was significantly increased during coexpression of Lck-YFP-N and ITGB1-YFP-C in Cos7 cells ( P <0.03 vs Lck alone and ITGB1 alone, n= 2 independent experiments, error bars represent ±s.d.). ( i ) Cell fluorescence intensity correlates to increasing YFP-N-LCK expression in Cos7 cells ( n= 3 independent experiments, y axis=log 10 , error bars represent ±s.d). ( j ) Active Lck binds directly to β1-integrin in a chemiluminescence binding assay using recombinant human proteins (Meso Scale Discovery). Representative signal measurements are shown for active Lck bound to β1-integrin, with saturating concentrations of active Lck and β1-integrin of 20 nM and 200 nM ( n= duplicate wells, error bars represent ±s.d). Non-specific binding (BSA) showed a negligible signal. Statistical significance was determined by two-tailed Student’s t -test. Full size image To confirm that Lck directly interacts with β1-integrin in a signalling complex, we utilized bimolecular fluorescence complementation (BiFC) to identify in vivo β1-integrin–Lck complex formation. BiFC constructs were generated containing the N-terminal fragment of YFP (amino acids (a.a.) 1–158) fused to the amino terminus of Lck and the C-terminal fragment of YFP (a.a. 159–235) fused to the carboxy terminus of β1-integrin. If the two YFP fragment-tagged proteins closely interact in vivo , they will recombine and produce a fluorescent signal that is not seen with expression of the individual YFP subunits alone [27] , [28] . Expression of YFP-N-Lck or ITGB1-YFP-C alone did not produce YFP fluorescence ( Fig. 1g ). Coexpression of both constructs induced a significant increase in YFP fluorescence, indicating that Lck and β1-integrin associate in vivo to form a signalling complex ( Fig. 1g , P <0.02). A positive correlation of average fluorescence intensity per cell to Lck-ITGB1 interaction was seen by transfecting increasing amounts of YFP-N-LCK with a constant amount of ITGB1-YFP-C ( Fig. 1i ). To assess direct Lck-ITGB1 binding affinity, we measured active Lck and ITGB1 interactions using recombinant human proteins in a ligand binding assay. Recombinant active Lck exhibited direct binding affinity to both 20 and 200 nM ITGB1 ( Fig. 1j ). Lck regulates paxillin and CrkII phosphorylation in SCs Paxillin is a primary molecular adaptor protein involved in integrin signalling [29] and coordinates the activation of multiple downstream signalling pathways, localizes to focal adhesion contacts, and stimulates lamellipodia formation and cytoskeletal rearrangement [30] . To elucidate the role of Lck signalling on paxillin and other downstream effector proteins of β1-integrin, we used a Lck inhibitor (A770041, Abbott Biochemicals) that specifically binds to the Lck active site at nanomolar concentrations and shows 8-, 60- and 300-fold specificity for Lck over Src kinase family members Lyn, Src and Fyn, respectively [31] , [32] . In RSC cultures, 500 nM Lck inhibitor does not inhibit Fyn, Src or Lyn ( Supplementary Fig. S2 ). RSCs seeded on laminin and treated with Lck inhibitor show a significant reduction in total levels of phospho(Y394)-Lck, phospho(Y118)-paxillin and phospho(Y221)-CrkII ( Fig. 2a , P =0.04, P <0.03 and P <0.001, respectively). Similarly, Lck downregulation by siRNA in RSCs ( Fig. 2b ) and lack of Lck in Lck −/− mouse SCs ( Fig. 2c ) results in a significant reduction in paxillin and CrkII phosphorylation on a laminin substrate. Furthermore, siRNA knockdown of β1-integrin results in considerable decreases in paxillin and CrkII phosphorylation ( Supplementary Fig. S1 ). The amount of activated paxillin (phospho-Y118) localized to the cell surface of lamellipodia is greatly reduced in RSC cultures seeded on a laminin substrate and treated with Lck inhibitor ( Fig. 2d ). To determine whether Lck inhibition has a similar effect on SCs interacting with axons, RSCs were seeded on DRG cultures and treated with Lck inhibitor for 3 days. The level of phospho(Y118)-paxillin was significantly reduced in cocultures treated with Lck inhibitor ( Fig. 2e , P <0.0001). Similarly, downregulation of Lck expression by siRNA before seeding on DRGs also leads to reduced paxillin phosphorylation ( Supplementary Fig. S1 ). A previous study had reported the association between Lck and paxillin in T cells, and that lack of Lck reduced the phosphorylation of paxillin in Lck-deficient T cells [33] . Here we show that recombinant active Lck binds directly to recombinant paxillin with the dissociation constant ( K D ) of 8.1 nM ( Fig. 2f ). 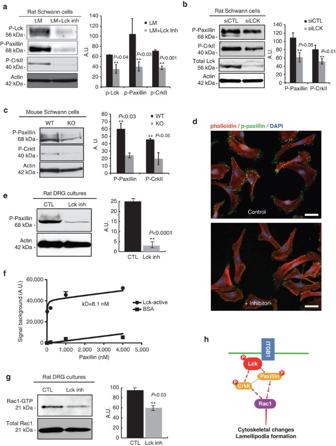Figure 2: Inhibition of Lck reduces paxillin and CrkII phosphorylation, and Rac-GTP levels in primary RSCs and SC-DRG cocultures. (a) RSCs seeded on laminin substrate were left untreated (LM) or treated (LM+Lck Inh) with 500 nM Lck inhibitor for 2 h. Lysates were analysed for phospho(Y394)-Lck, phospho(Y118)-paxillin, phospho(Y221)-CrkII and actin as a loading control. Treatment with Lck inhibitor significantly reduced the phosphorylation levels of Lck, paxillin and CrkII (graph shows densitometric quantification from three independent experiments, error bars represent ±s.d.). (b) Lck expression was downregulated with siRNA for 3 days then cells were seeded on laminin substrate for 3.5 h before lysis. Lysates were analysed as in (a). Lck downregulation significantly reduced the phosphorylation of paxillin and CrkII (n=2 independent experiments, error bars represent ±s.d.). (c) Mouse SCs purified from wild-type and Lck−/−mice were seeded on laminin substrate for 3.5 h, then lysates were analysed as ina. Paxillin and CrkII phosphorylation were significantly reduced in Lck−/−SCs (n=2 independent experiments, error bars represent ±s.d.). (d) SCs were stained for phalloidin-rhodamine and phospho(Y118)-paxillin to identify lamellipodia and active paxillin. Paxillin phosphorylation was reduced in Lck inhibitor-treated cultures as compared with control in both radial and axial lamellipodia. (e) Schwann cell-neuron cocultures were treated without (CTL) or with 500 nM Lck inhibitor (Lck inh) for 3 days then lysates were analysed for phospho(Y118)-paxillin. Phospho-paxillin was significantly reduced in cocultures treated with Lck inhibitor for 3 days (P<0.0001, 10 cultures per sample,n=5 experiments, error bars represent ±s.d.). (f) Representative saturation plot for active Lck bound to paxillin is shown (n=duplicate wells, error bars represent ±s.d.). TheKDvalue for paxillin-active Lck binding was 8.1 nM, as determined by nonlinear curve fitting using GraphPad Prism 6.0 software. (g) Schwann cell-DRG cocultures were treated without (CTL) or with Lck inhibitor for 3 days then lysates were analysed for Rac-GTP using a Rac1-GTP pull-down assay. Rac1-GTP was significantly reduced following treatment with Lck inhibitor (P<0.03, 10 cultures per sample,n=3 independent experiments). Total Rac1 remains unchanged. (h) Schematic model of the Lck mediated signalling pathway that regulates cytoskeletal changes and migration in SCs. Scale bars represent 50 μm. Statistical significance was determined by two-tailed Student’st-test. Figure 2: Inhibition of Lck reduces paxillin and CrkII phosphorylation, and Rac-GTP levels in primary RSCs and SC-DRG cocultures. ( a ) RSCs seeded on laminin substrate were left untreated (LM) or treated (LM+Lck Inh) with 500 nM Lck inhibitor for 2 h. Lysates were analysed for phospho(Y394)-Lck, phospho(Y118)-paxillin, phospho(Y221)-CrkII and actin as a loading control. Treatment with Lck inhibitor significantly reduced the phosphorylation levels of Lck, paxillin and CrkII (graph shows densitometric quantification from three independent experiments, error bars represent ±s.d.). ( b ) Lck expression was downregulated with siRNA for 3 days then cells were seeded on laminin substrate for 3.5 h before lysis. Lysates were analysed as in ( a ). Lck downregulation significantly reduced the phosphorylation of paxillin and CrkII ( n= 2 independent experiments, error bars represent ±s.d.). ( c ) Mouse SCs purified from wild-type and Lck −/− mice were seeded on laminin substrate for 3.5 h, then lysates were analysed as in a . Paxillin and CrkII phosphorylation were significantly reduced in Lck −/− SCs ( n= 2 independent experiments, error bars represent ±s.d.). ( d ) SCs were stained for phalloidin-rhodamine and phospho(Y118)-paxillin to identify lamellipodia and active paxillin. Paxillin phosphorylation was reduced in Lck inhibitor-treated cultures as compared with control in both radial and axial lamellipodia. ( e ) Schwann cell-neuron cocultures were treated without (CTL) or with 500 nM Lck inhibitor (Lck inh) for 3 days then lysates were analysed for phospho(Y118)-paxillin. Phospho-paxillin was significantly reduced in cocultures treated with Lck inhibitor for 3 days ( P <0.0001, 10 cultures per sample, n= 5 experiments, error bars represent ±s.d.). ( f ) Representative saturation plot for active Lck bound to paxillin is shown ( n= duplicate wells, error bars represent ±s.d.). The K D value for paxillin-active Lck binding was 8.1 nM, as determined by nonlinear curve fitting using GraphPad Prism 6.0 software. ( g ) Schwann cell-DRG cocultures were treated without (CTL) or with Lck inhibitor for 3 days then lysates were analysed for Rac-GTP using a Rac1-GTP pull-down assay. Rac1-GTP was significantly reduced following treatment with Lck inhibitor ( P <0.03, 10 cultures per sample, n= 3 independent experiments). Total Rac1 remains unchanged. ( h ) Schematic model of the Lck mediated signalling pathway that regulates cytoskeletal changes and migration in SCs. Scale bars represent 50 μm. Statistical significance was determined by two-tailed Student’s t -test. Full size image Rac-GTP activation during SC ensheathment of axons Rac1 has been identified as a downstream target of paxillin and a critical mediator of β1-integrin signalling that regulates the formation of radial lamellipodia in SCs [21] . To determine whether Lck signalling is involved in the activation of Rac1 in SCs during axonal sorting, SC-neuron cocultures were treated with Lck inhibitor for 3 days. Inhibition of Lck in SC-neuron cocultures resulted in a significant reduction in Rac-GTP levels ( Fig. 2g , P <0.03). These results suggest that Lck signalling regulates paxillin phosphorylation at the Y118 active site, which subsequently affects Rac1-GTP formation, leading to a decreased formation of radial lamellipodia (shown below). This pathway is schematically represented in Fig. 2h . Lck regulates the formation of radial lamellipodia Laminin induces formation of axial and radial lamellipodia in SCs [13] , [34] . To determine the effect of Lck inhibition on lamellipodia formation, RSCs were seeded on a laminin substrate then treated with Lck inhibitor or dimethylsulphoxide (DMSO). The number of lamellipodia formed by inhibitor-treated cells was significantly lower than in untreated cells ( Fig. 3a–c , P <0.0003). Time-lapse photography of RSCs on a laminin substrate showed a reduction in the extension and retraction of lamellipodia (arrowheads) in inhibitor-treated cultures as compared with control ( Fig. 3e ; Supplementary Movies 1 and 2 ). Lck inhibition had no effect on axial lamellipodia ( Fig. 3e ; Supplementary Movies 1 and 2 ) and SC morphology or spreading on collagen IV, fibronectin or poly- L -lysine ( Supplementary Fig. S3 ). 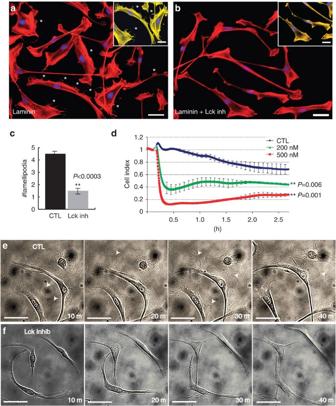Figure 3: Inhibition of Lck reduces the formation of radial lamellipodia in SCs. RSCs seeded on a laminin substrate were allowed to attach for 1.5 h, then were left untreated (a) or treated (b) with 500 nM Lck inhibitor for 2 h. Cultures were fixed and stained for phalloidin-rhodamine to identify lamellipodia (asterisks). Insets show magnified images of SCs pseudo-coloured yellow using Photoshop to represent the loss of radial lamellipodia (asterisks) after treatment with Lck inhibitor. (c) Numbers of radial lamellipodia per cell seeded on a laminin substrate were counted (30 cells per well,n=4 from two independent experiments, error bars represent ±s.d.). Treatment with Lck inhibitor significantly reduced the number of radial lamellipodia per cell on a laminin substrate (P<0.0003). (d) RSCs were seeded onto a laminin-coated xCELLigence E-plate and allowed to attach for 2 h. Cell spreading was monitored every 15 s following addition of DMSO (CTL), 200 nM Lck inhibitor or 500 nM Lck inhibitor. Addition of Lck inhibitor induced an immediate retraction of cell processes as compared with DMSO treated cultures (CTL line in graph). A slight increase in cell index, indicating cell spreading, was seen after the acute phase of treatment but overall the cell index remained significantly decreased after 2 h (n=4,P<0.006 (200 nM) andP<0.001 (500 nM) by Student’st-test, error bars represent ±s.d.). (e,f) RSCs were seeded on laminin substrate and live cell imaging was performed with images acquired every 2 min using a Zeiss Axiovert microscope equipped with the AxioVision Software. Dynamic extension and retraction of radial lamellipodia were seen in control cultures (e, arrowheads) while only initial retraction and no extensions of radial lamellipodia were seen during Lck inhibition (f). Scale bars represent 50 μm. Figure 3: Inhibition of Lck reduces the formation of radial lamellipodia in SCs. RSCs seeded on a laminin substrate were allowed to attach for 1.5 h, then were left untreated ( a ) or treated ( b ) with 500 nM Lck inhibitor for 2 h. Cultures were fixed and stained for phalloidin-rhodamine to identify lamellipodia (asterisks). Insets show magnified images of SCs pseudo-coloured yellow using Photoshop to represent the loss of radial lamellipodia (asterisks) after treatment with Lck inhibitor. ( c ) Numbers of radial lamellipodia per cell seeded on a laminin substrate were counted (30 cells per well, n= 4 from two independent experiments, error bars represent ±s.d.). Treatment with Lck inhibitor significantly reduced the number of radial lamellipodia per cell on a laminin substrate ( P <0.0003). ( d ) RSCs were seeded onto a laminin-coated xCELLigence E-plate and allowed to attach for 2 h. Cell spreading was monitored every 15 s following addition of DMSO (CTL), 200 nM Lck inhibitor or 500 nM Lck inhibitor. Addition of Lck inhibitor induced an immediate retraction of cell processes as compared with DMSO treated cultures (CTL line in graph). A slight increase in cell index, indicating cell spreading, was seen after the acute phase of treatment but overall the cell index remained significantly decreased after 2 h ( n= 4, P <0.006 (200 nM) and P <0.001 (500 nM) by Student’s t -test, error bars represent ±s.d.). ( e , f ) RSCs were seeded on laminin substrate and live cell imaging was performed with images acquired every 2 min using a Zeiss Axiovert microscope equipped with the AxioVision Software. Dynamic extension and retraction of radial lamellipodia were seen in control cultures ( e , arrowheads) while only initial retraction and no extensions of radial lamellipodia were seen during Lck inhibition ( f ). Scale bars represent 50 μm. Full size image To further analyse the effect of Lck on cell spreading/lamellipodia formation, we seeded RSCs on laminin-coated wells and assessed cell spreading with the xCELLigence System (Roche) that measures total surface area covered by cell membrane by detecting the electrical impedance, using a microelectronic biosensor technology [35] . Following addition of Lck inhibitor, but not DMSO alone, the cell index dropped dramatically, indicating that many cell processes immediately retracted ( Fig. 3d ). The slow rise in cell index over time suggests some recovery in the Lck inhibitor-treated wells, but a significant reduction in the cell index remained after 2 h of 200- and 500-nM inhibitor treatment ( P <0.006 and P <0.001, respectively), corroborating the reduction in radial lamellipodia following Lck inhibition for 2 h (see Fig. 3c ). Inhibition of Lck slows the rate of SC migration As inhibition of Lck signalling has a dramatic effect on radial lamellipodia extension and retraction, we investigated whether Lck may also function to regulate the extension and migration of SCs along axons. Live imaging was conducted on green fluorescent protein-expressing RSCs seeded on rat DRG cultures. Cultures were treated with Lck inhibitor or DMSO for 24 h and imaged every 10 min ( Fig. 4a ; Supplementary Movies 3 and 4 ). Lck inhibition severely inhibited RSC extension and migration along axons, while local axial exploration of their environment was maintained ( Fig. 4a ; Supplementary Movies 3 and 4 ). In control cultures, approximately half of the cells migrated over 25 μm h −1 . Conversely, over half of the inhibitor-treated cells did not migrate at all, or migrated <10 μm h −1 and only 18% of the cells were able to reach a migration rate >25 μm h −1 ( Fig. 4b ). These results indicate that Lck mediates extension and longitudinal migration of SCs along an axon in addition to the β1-integrin-mediated radial lamellipodia formation necessary for radial sorting. 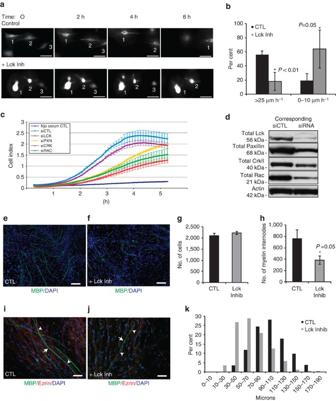Figure 4: Inhibition of Lck activity slows SC migration on axons and inhibits myelination. (a,b) GFP-transfected RSCs on DRG axons were treated with Lck inhibitor (500 nM) or DMSO alone (CTL) and the cultures were imaged every 10 min for 24 h. The migration rate is shown as the percentage of highly migrating (>25 μm h−1; cells 1–3 on the upper frames), slow migrating cells (0–10 μm h−1; cell 3 on the lower frames) or stationary cells (cells 1–2 on the lower frames). Lck inhibition significantly reduced the number of actively migrating cells (n=30,P<0.01, error bars represent ±s.d.), while slow or stationary cells were significantly increased (P=0.05, ±s.d.). (c) RSCs were transfected with siRNAs against Lck, paxillin, Crk, Rac or a non-targeting siRNA. Three days post transfection, the cell migration was recorded on an xCELLigence CIM plate. Reduced expression of Lck, paxillin and Rac significantly decreased RSC migration rate during 2–4 h as compared with control (P=0.01,P=0.03 andP=0.02, respectively,n=3 independent experiments, error bars represent ±s.d.). (d) Levels of Lck, paxillin, CrkII, Rac and actin as a loading control in RSCs used inc. SC-neuron cocultures were treated continuously (e) without or (f) with 500 nM Lck inhibitor for 13 days after the induction of myelination. Cultures were immunostained for MBP (green) and 4′,6-diamidino-2-phenylindole (DAPI; blue). (g,h) Myelin internodes were counted from ten × 10 fields per culture. Treatment with Lck inhibitor significantly reduced the number of myelin internodes (h,P=0.05,n=7 from two independent experiments, error bars represent ±s.e.m.), without affecting total cell numbers (g). SC-neuron cocultures were treated as above then fixed and immunostained for MBP, ezrin and DAPI. Ezrin staining was localized to the nodes in both control (i) and inhibitor-treated (j) cultures and each internode is associated with one nucleus, indicating that Lck inhibition results in shorter, but mature internodes. Arrows indicate an internode between two ezrin-positive nodes (arrow heads). (k) The length of myelin internodes (~100 internodes per culture) was measured and the size distribution is shown. The majority of internodes in Lck inhibitor-treated cultures are shorter than in control cultures (n=7 from two experiments). Scale bars represent 50 μm. Statistical significance was determined by two-tailed Student’st-test. Figure 4: Inhibition of Lck activity slows SC migration on axons and inhibits myelination. ( a , b ) GFP-transfected RSCs on DRG axons were treated with Lck inhibitor (500 nM) or DMSO alone (CTL) and the cultures were imaged every 10 min for 24 h. The migration rate is shown as the percentage of highly migrating (>25 μm h −1 ; cells 1–3 on the upper frames), slow migrating cells (0–10 μm h −1 ; cell 3 on the lower frames) or stationary cells (cells 1–2 on the lower frames). Lck inhibition significantly reduced the number of actively migrating cells ( n= 30, P <0.01, error bars represent ±s.d. ), while slow or stationary cells were significantly increased ( P =0.05, ±s.d.). ( c ) RSCs were transfected with siRNAs against Lck, paxillin, Crk, Rac or a non-targeting siRNA. Three days post transfection, the cell migration was recorded on an xCELLigence CIM plate. Reduced expression of Lck, paxillin and Rac significantly decreased RSC migration rate during 2–4 h as compared with control ( P =0.01, P =0.03 and P =0.02, respectively, n= 3 independent experiments, error bars represent ±s.d.). ( d ) Levels of Lck, paxillin, CrkII, Rac and actin as a loading control in RSCs used in c . SC-neuron cocultures were treated continuously ( e ) without or ( f ) with 500 nM Lck inhibitor for 13 days after the induction of myelination. Cultures were immunostained for MBP (green) and 4′,6-diamidino-2-phenylindole (DAPI; blue). ( g , h ) Myelin internodes were counted from ten × 10 fields per culture. Treatment with Lck inhibitor significantly reduced the number of myelin internodes ( h , P =0.05, n= 7 from two independent experiments, error bars represent ±s.e.m. ), without affecting total cell numbers ( g ). SC-neuron cocultures were treated as above then fixed and immunostained for MBP, ezrin and DAPI. Ezrin staining was localized to the nodes in both control ( i ) and inhibitor-treated ( j ) cultures and each internode is associated with one nucleus, indicating that Lck inhibition results in shorter, but mature internodes. Arrows indicate an internode between two ezrin-positive nodes (arrow heads). ( k ) The length of myelin internodes (~100 internodes per culture) was measured and the size distribution is shown. The majority of internodes in Lck inhibitor-treated cultures are shorter than in control cultures ( n= 7 from two experiments). Scale bars represent 50 μm. Statistical significance was determined by two-tailed Student’s t -test. Full size image To assess the contribution of Lck, paxillin, CrkII and Rac to the migration rate of RSCs, a transwell migration assay was conducted following siRNA downregulation of the respective proteins ( Fig. 4c ). Downregulation of Lck, paxillin and Rac significantly decreased the rate of RSC migration (calculated from hours 2–4) as compared with control ( P =0.01, P =0.03 and P =0.02, respectively), indicating an essential role of these kinases for RSC migration. The greatest reduction is seen following Lck downregulation (0.364 h −1 ) as compared with control (0.896 h −1 ). On the basis of these data, activation of CrkII does not have a central role in the regulation of SC migration but rather is an intermediate of the Lck signalling pathway. Lck regulates the number and length of myelin internodes To determine the effect of Lck inhibition on myelination, cocultures were treated with 500 nM Lck inhibitor at the time of seeding and continuously during ascorbate treatment for 10–14 days. Treatment with Lck inhibitor significantly reduced the number of myelin internodes formed compared with control cocultures ( Fig. 4e–h , P =0.05). The length of myelin internodes was measured, and a significant shift to shorter myelin internodes (30–70 μm) was found after Lck inhibition compared with untreated cocultures (70–110 μm) ( Fig. 4k ). To confirm that the role of Lck signalling on myelination was due to a SC effect and not an axonal effect, siRNA knockdown was used to reduce Lck expression in SCs before seeding on DRG cultures. The number of myelin internodes in Lck knockdown cultures was significantly reduced as compared with control cultures ( Supplementary Fig. S4 ; P <0.029). Mouse DRG-SC cocultures were also used to confirm that wild-type (WT) mouse SCs seeded on Lck −/− axons were able to myelinate at the same level as WT SCs seeded on WT axons ( Supplementary Fig. S4 ). To investigate whether the shorter internodes were due to incomplete myelination by one SC, which occurs during ROCK inhibition [36] , cultures were stained for myelin basic protein (MBP) and ezrin to identify mature nodes. The shorter internodes formed in inhibitor-treated cultures did have ezrin localized at the nodes, with a nucleus associated with each myelin internode (arrows) as in control cultures ( Fig. 4i ). These results indicate that the SCs form a complete mature myelin sheath but do not extend and wrap to the same length as untreated SCs, supporting the effects of Lck inhibition on SC axial extension along axons, as shown in Fig. 4a . Loss of Lck slows SC migration and delays myelination To determine whether inhibition of Lck signalling will slow the progression of SCs along extending axons, we used mouse DRG explants with specific culture conditions to promote axon outgrowth before the migration of SCs out of the explant (see Supplementary Methods ). Lck inhibitor treatment was started before any mouse SC migration out of the explant (day 4 in culture) and the migration distance of endogenous SCs from the explant was measured after 6 days of inhibitor treatment. Inhibition of Lck significantly reduced the distance that SCs were able to migrate along the axons ( P <0.02, Fig. 5a ). Axon outgrowth was only slightly reduced in inhibitor-treated explants, but was not significant (data not shown). 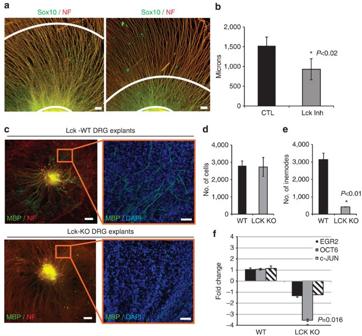Figure 5: Lck inhibition impedes migration of mouse SCs along axons and Lck−/−DRG explants show decreased myelination. (a) Mouse DRG explants were isolated and cultured to enhance axonal outgrowth before SC migration out of the explant (seeSupplementary Methods). Cultures were treated with DMSO (CTL) or 500 nM Lck inhibitor beginning at day 4 after seeding. Treatment was continuous for 6 days, then cultures were fixed and immunostained for Sox10, neurofilament and 4′,6-diamidino-2-phenylindole (DAPI). Distance from the explant to the edge of the migrated Sox10-positive mouse SCs (white concentric lines) was measured (eight measurements per explant). (b) Lck inhibition significantly reduced the distance that Sox10-positive SCs migrated along the axons (P<0.02,n=4 from two independent experiments, error bars represent ±s.d.). (c) DRG explant cultures from WT or Lck−/−mice were cultured for 17 days to allow complete population of the explant with endogenous SCs, then ascorbic acid was added to the media for 11 days to induce myelination. The cultures were fixed and immunostained for MBP (green), neurofilament (red) and DAPI (blue). Left panels represent compiled mosaic images covering the whole explant culture and the insets (right panels) represent magnified images from the mosaic to depict myelin internodes. (d) Quantification of DAPI-positive nuclei in Lck−/−and WT explants showed no difference in the number of SCs. (e) Quantification of myelin internodes in Lck−/−and WT DRG explants. The number of myelin internodes was significantly reduced in Lck−/−DRG explants (n=2,P<0.01, error bars represent ±s.d.). (f) RNA was isolated from WT and Lck−/−DRG explants 11 days after initiation of myelination (n=2, three cultures per sample). Quantitative real-time PCR (Applied Biosystems) for Egr2, Oct-6, c-Jun and GAPDH mRNA was conducted and the relative RNA abundance, normalized to GAPDH, was determined by the 2−ΔΔCtmethod. The fold change in mRNA in Lck−/−cultures as compared with WT cultures is shown. The level of Oct-6 mRNA was significantly reduced in Lck−/−cultures as compared with WT (P=0.016, error bars represent ±s.d.). No significant change in Egr2 or c-Jun expression was seen in Lck−/−explants. Scale bars represent 100 μm (a,cinset), 500 μm (c). Statistical significance was determined by two-tailed Student’st-test. Figure 5: Lck inhibition impedes migration of mouse SCs along axons and Lck −/− DRG explants show decreased myelination. ( a ) Mouse DRG explants were isolated and cultured to enhance axonal outgrowth before SC migration out of the explant (see Supplementary Methods ). Cultures were treated with DMSO (CTL) or 500 nM Lck inhibitor beginning at day 4 after seeding. Treatment was continuous for 6 days, then cultures were fixed and immunostained for Sox10, neurofilament and 4′,6-diamidino-2-phenylindole (DAPI). Distance from the explant to the edge of the migrated Sox10-positive mouse SCs (white concentric lines) was measured (eight measurements per explant). ( b ) Lck inhibition significantly reduced the distance that Sox10-positive SCs migrated along the axons ( P <0.02, n= 4 from two independent experiments, error bars represent ±s.d.). ( c ) DRG explant cultures from WT or Lck −/− mice were cultured for 17 days to allow complete population of the explant with endogenous SCs, then ascorbic acid was added to the media for 11 days to induce myelination. The cultures were fixed and immunostained for MBP (green), neurofilament (red) and DAPI (blue). Left panels represent compiled mosaic images covering the whole explant culture and the insets (right panels) represent magnified images from the mosaic to depict myelin internodes. ( d ) Quantification of DAPI-positive nuclei in Lck −/− and WT explants showed no difference in the number of SCs. ( e ) Quantification of myelin internodes in Lck −/− and WT DRG explants. The number of myelin internodes was significantly reduced in Lck −/− DRG explants ( n= 2, P <0.01, error bars represent ±s.d.). ( f ) RNA was isolated from WT and Lck −/− DRG explants 11 days after initiation of myelination ( n= 2, three cultures per sample). Quantitative real-time PCR (Applied Biosystems) for Egr2, Oct-6, c-Jun and GAPDH mRNA was conducted and the relative RNA abundance, normalized to GAPDH, was determined by the 2 −ΔΔCt method. The fold change in mRNA in Lck −/− cultures as compared with WT cultures is shown. The level of Oct-6 mRNA was significantly reduced in Lck −/− cultures as compared with WT ( P =0.016, error bars represent ±s.d.). No significant change in Egr2 or c-Jun expression was seen in Lck −/− explants. Scale bars represent 100 μm ( a , c inset), 500 μm ( c ). Statistical significance was determined by two-tailed Student’s t -test. Full size image To determine whether Lck −/− SCs are defective in myelination similar to pharmacological inhibition of Lck (see Fig. 4e–h ), we cultured WT and Lck −/− DRG explants for 17 days to allow for equal population of axons with endogenous mouse SCs. Ascorbate was then added to the media for 11 days. Myelin internode formation was greatly reduced in Lck −/− cultures, while total numbers of SCs remained similar ( Fig. 5c–e , P <0.01). Loss of Lck affects the expression levels of Oct-6 Lck signalling through its role in the regulation of radial lamellipodia formation and migration in SCs may also affect the expression of genes that mediate the myelination programme. To examine this, we analysed the major transcriptional regulators of myelination (c-jun, Oct-6 and Egr2) in WT and Lck −/− DRG explants undergoing myelination. mRNA levels of Egr2 and c-Jun were not significantly different, but Oct-6 mRNA in Lck −/− cultures was decreased 3-fold as compared with WT cultures ( Fig. 5f , P =0.016). Oct-6 expression levels rise in promyelinating SCs as they form a 1:1 ratio with axons and before Egr2 and myelin gene expression, suggesting that fewer Lck −/− SCs have correctly sorted axons than in WT SCs. Expression of Oct-6 in the mouse sciatic nerve transiently peaks in the first postnatal week while most of the SCs are at the ‘promyelinating’ stage of development [37] . We analysed the expression levels of Oct-6 and Egr2 protein in P5 mouse sciatic nerves from WT and Lck −/− animals. Oct-6 protein levels were significantly reduced in Lck −/− nerves as compared with WT nerves ( Fig. 6a , P =0.003). In contrast, Egr2 protein levels were unchanged in the Lck −/− nerves at postnatal day 5 ( Fig. 6a ). These results suggest that defects in cytoskeletal dynamics and SC migration ultimately affect axonal sorting and the upregulation of Oct-6 protein levels in promyelinating SCs. Lck −/− mice did not show changes in expression of ErbB2, ErbB3 or Nrg1 ( Supplementary Fig. S5 ), indicating that the neuregulin signalling pathway is maintained in P5 sciatic nerves. 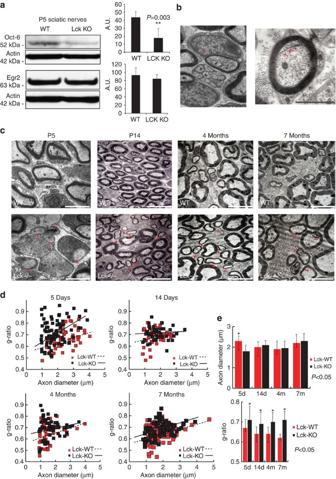Figure 6: Lck−/−mice exhibit characteristic pathology of the PNS. (a) Sciatic nerves from 5-day WT and Lck−/−mice were isolated and lysates were analysed for Oct-6 and Egr2 protein expression levels. Oct-6 expression levels are significantly lower in Lck−/−sciatic nerves as compared with WT sciatic nerves (P=0.003,n=5, four nerves per sample, error bars represent ±s.d.). Conversely, no significant differences in Egr2 expression are seen. (b) Left panel shows an Lck−/−SC forming compact myelin around a bundle that contains several small diameter axons suggesting an abnormal sorting process (arrow). Scale bar shows × 4,000 magnification. Right panel shows a P14 sciatic nerve of Lck−/−mice with intimate interdigitations between the inner aspect of the SC and the axon (arrows). Scale bar denotes × 6,000 magnification. (c) Sciatic nerves from Lck−/−mice show delay in myelination as compared with their WT littermates. Arrows (first panel bottom row) show SCs at P5 that have established a 1:1 relationship with large-diameter axons but have not initiated the myelination programme. Arrows in the remaining bottom panels denote several axons with thin myelin sheaths as compared with their WT littermates at 14 days, 4 months and 7 months. Arrowhead in the bottom right panel shows representative example of interleaved myelin folding in 7-month Lck−/−mice. Scale bars denote × 4,000 magnification. (d) Quantification of the g-ratios versus axon diameters of myelinated axons between Lck−/−and WT littermates at P5, P14, 4 and 7 months shows an abnormal distribution of g-ratios in Lck−/−mice. (e) Quantification of the axon diameters and the g-ratios between sciatic nerves from Lck−/−mice and their WT littermates in various time intervals (5days, 14 days, 4 months and 7 months). Axon diameters and g-ratios were quantified using sciatic nerves from two animals in each group and are plotted as average±s.d. Statistical significance was determined by two-tailed Student’st-test. Figure 6: Lck −/− mice exhibit characteristic pathology of the PNS. ( a ) Sciatic nerves from 5-day WT and Lck −/− mice were isolated and lysates were analysed for Oct-6 and Egr2 protein expression levels. Oct-6 expression levels are significantly lower in Lck −/− sciatic nerves as compared with WT sciatic nerves ( P =0.003, n= 5, four nerves per sample, error bars represent ±s.d.). Conversely, no significant differences in Egr2 expression are seen. ( b ) Left panel shows an Lck −/− SC forming compact myelin around a bundle that contains several small diameter axons suggesting an abnormal sorting process (arrow). Scale bar shows × 4,000 magnification. Right panel shows a P14 sciatic nerve of Lck −/− mice with intimate interdigitations between the inner aspect of the SC and the axon (arrows). Scale bar denotes × 6,000 magnification. ( c ) Sciatic nerves from Lck −/− mice show delay in myelination as compared with their WT littermates. Arrows (first panel bottom row) show SCs at P5 that have established a 1:1 relationship with large-diameter axons but have not initiated the myelination programme. Arrows in the remaining bottom panels denote several axons with thin myelin sheaths as compared with their WT littermates at 14 days, 4 months and 7 months. Arrowhead in the bottom right panel shows representative example of interleaved myelin folding in 7-month Lck −/− mice. Scale bars denote × 4,000 magnification. ( d ) Quantification of the g-ratios versus axon diameters of myelinated axons between Lck −/− and WT littermates at P5, P14, 4 and 7 months shows an abnormal distribution of g-ratios in Lck −/− mice. ( e ) Quantification of the axon diameters and the g-ratios between sciatic nerves from Lck −/− mice and their WT littermates in various time intervals (5days, 14 days, 4 months and 7 months). Axon diameters and g-ratios were quantified using sciatic nerves from two animals in each group and are plotted as average±s.d. Statistical significance was determined by two-tailed Student’s t -test. Full size image Lck −/− mice exhibit defects during PNS myelination The Lck −/− mice are fertile, viable and show no macroscopic defect of the PNS. They have a pronounced thymic atrophy and complete lack of mature T cells [38] . To examine the effects of the loss of Lck expression during the development and maturation of the PNS in the Lck −/− mice, we utilized electron microscopy to assess in vivo SC maturation. Electron microscopy of the sciatic nerves revealed that the ensheathment of non-myelinated axons is defective in P14 Lck −/− mice ( Fig. 6b ). In particular, we observed intimate interdigitations between the inner aspect of the SC and the myelinated axon ( Fig. 6b , arrows) and abnormal myelination around bundles of several axons ( Fig. 6b , arrow), which implies an abnormal sorting process. However, this is a transient phenotype as we did not observe sorting problems in adult mice ( Fig. 6c ). Moreover, Lck −/− mice exhibit a delay in myelination ( Fig. 6c , arrows) and overall thinner myelin sheaths. In fact, quantification of axon diameters and g-ratios between WT and Lck −/− mice over a period of 7 months shows that Lck −/− mice exhibit progressively thinner myelin sheaths (higher g-ratios) while the axon diameters are not affected ( Fig. 6d , n= 2). We believe that the difference in axon diameter in P5 sciatic nerves only ( Fig. 6e ), represents a reflection of the developmental delay in myelination and overall delayed maturation of the myelinated axons in Lck −/− mice. Finally, we observed myelin outfoldings in cross-sections of sciatic nerves ( Fig. 7a ). These myelin structures appeared more often in Lck −/− mice as compared with WT mice and became more prominent as the mice got older ( Fig. 7a ). The aberrant myelin membranes were either facing away from the axon cylinder or towards the axon ( Fig. 7c ), and electron microscopic analysis of longitudinal sciatic nerve sections (2 months) of Lck −/− mice revealed that the myelin abnormalities originate from the paranodal regions ( Fig. 7c ). This myelin pathology is present in various models of peripheral neuropathies and especially resembles the myelin pathology observed in Mtmr2 m/m mice (model for CMT4B1) [39] . However, as in the case of Mtmr2 mice, the exact role of these myelin abnormalities in Lck −/− mice is not clear yet. 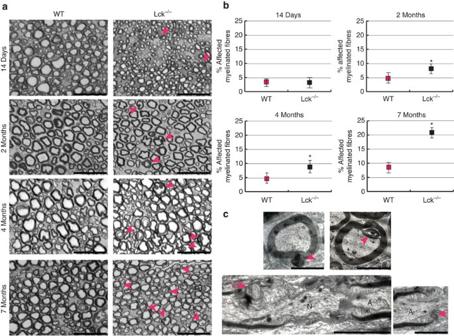Figure 7: Lck−/−mice exhibit abnormal myelin folding. (a) Time course analysis of sciatic nerves. Sciatic nerve cross-sections of WT (left panels top to bottom) and Lck−/−(right panels top to bottom) mice. The morphology of myelin was compared at the age of 14 days (upper two panels), 2 months (second row of panels), 4 months (third row) and 7 months (last row). Two animals were analysed per age and phenotype, and representative pictures are shown. Examples of affected axons with aberrant myelin loops in Lck−/−mice are marked with arrowheads. Scale bar for all panels: 25 μm. (b) Quantification of aberrant myelin loops during the time course (14 days–7 months). For each time interval the sciatic nerves from two mice were isolated and semithin sections were quantified. The number of affected myelin fibres increases with age in Lck−/−mice. The results are presented as average±s.d. and statistical significance is denoted as *P<0.05. (c) Electron microscopic analysis of sciatic nerves from Lck−/−mice shows abnormal myelin outfoldings (upper left panel) and infoldings (upper right) in large-diameter axons (marked by arrowheads). Longitudinal electron microscope sections show aberrant myelin loops at the paranodal region of Lck−/−mice (bottom panels). Myelin loops are marked with an arrow. A, axon; N, node. Scale bars, 2 μm. Statistical significance was determined by two-tailed Student’st-test. Figure 7: Lck −/− mice exhibit abnormal myelin folding. ( a ) Time course analysis of sciatic nerves. Sciatic nerve cross-sections of WT (left panels top to bottom) and Lck −/− (right panels top to bottom) mice. The morphology of myelin was compared at the age of 14 days (upper two panels), 2 months (second row of panels), 4 months (third row) and 7 months (last row). Two animals were analysed per age and phenotype, and representative pictures are shown. Examples of affected axons with aberrant myelin loops in Lck −/− mice are marked with arrowheads. Scale bar for all panels: 25 μm. ( b ) Quantification of aberrant myelin loops during the time course (14 days–7 months). For each time interval the sciatic nerves from two mice were isolated and semithin sections were quantified. The number of affected myelin fibres increases with age in Lck −/− mice. The results are presented as average±s.d. and statistical significance is denoted as * P <0.05. ( c ) Electron microscopic analysis of sciatic nerves from Lck −/− mice shows abnormal myelin outfoldings (upper left panel) and infoldings (upper right) in large-diameter axons (marked by arrowheads). Longitudinal electron microscope sections show aberrant myelin loops at the paranodal region of Lck −/− mice (bottom panels). Myelin loops are marked with an arrow. A, axon; N, node. Scale bars, 2 μm. Statistical significance was determined by two-tailed Student’s t -test. Full size image The laminin/integrin and laminin/dystroglycan signalling pathways between SCs and the basal lamina converge with neuregulin/ErbB2/3 signalling between axons and SCs to direct the proliferation and radial sorting of axon bundles to produce the 1:1 ratio of SC:axon required for myelination. In this study, we identify Lck as a novel signalling component that mediates the propagation of β1-integrin signalling in SCs. Lck regulates the cytoskeletal rearrangement necessary for radial lamellipodia formation, which is required for radial sorting and myelination in the PNS. Lck signalling also facilitates extension and migration of SCs along axons. Lck is localized in a complex with β1-integrin and is upstream of paxillin and CrkII phosphorylation, and the upregulation of Rac1-GTP levels. Although other SFKs are well described as essential components of ECM–cell adhesion and migration pathways in glial cells [25] , [26] , this is the first report of a role for Lck kinase in laminin/β1-integrin signalling pathway in non-lymphocyte tissue. It is known that Fyn associates with the ITGB1–FAK–paxillin complex in late-differentiating SC-DRG cultures, in contrast to the early effect of Lck on paxillin phosphorylation [29] . Interestingly, Src kinase is involved in the p75 NTR -mediated inhibition of migration and promotion of myelination [40] . The role of SFKs therefore can have opposing effects on migration and myelination, which indicates that association with different receptor signalling complexes may define this role. Recently, a study showed that PP2, a general SFK inhibitor, leads to decreased myelination in SC-DRG cocultures, shorter internodes, and decreased Egr2 protein levels [41] . The results of our study indicate that it is the inhibition of Lck and not the inhibition of Fyn, Src or Lyn, which mediates the PP2 effects on myelination and shortened internodes. In this study, we have utilized Lck-specific siRNAs, a highly specific Lck inhibitor, A770041 (Abbott) [31] , [32] and Lck −/− mice. With this high degree of specificity, and by using an antibody specific to the phosphorylated active site of Lck, we are able to demonstrate the unique function of endogenous Lck kinase activity in SCs. Analysis of Lck −/− sciatic nerve and DRG explant cultures revealed that loss of Lck results in a delay in SC migration, axonal sorting and myelination, which is likely due to defective β1-integrin signalling to induce radial lamellipodia formation and SC migration. The laminin receptor, α6β1 integrin, is expressed in immature SCs and conditional deletion of β1-integrin in immature SCs inhibits the process of axonal sorting [16] , [17] , [42] . SC-specific deletion of the γ1 subunit of laminin results in a similar inhibition of axonal sorting by SCs [13] , [34] . In addition, the lack of laminin signalling inhibits SC process extension on axons, which is not seen in the β1-integrin null SCs. The variations in KO phenotype suggest that the loss of laminins affects β1-integrin signalling as well as other receptor function such as ErbB2/3 (ref. 14 ). Our data show that loss of Lck results in defects found in both laminin and β1-integrin KO SCs, but only transiently delays the onset of axonal sorting and myelination while it causes thinner myelination in older animals. Hence, we describe Lck as one of the downstream effectors of laminin/β1-integrin signalling, and pinpoint specific signalling cascades responsible for the cytoskeletal rearrangement initiated by laminin/β1-integrin signalling. The essential role for Lck in the formation of lamellipodia was demonstrated by the dramatic retraction of SC processes following Lck inhibition on a laminin substrate ( Fig. 3 ; Supplementary Fig. S3 ). The dynamic changes in cell adhesion and cytoskeletal reorganization required in the formation of lamellipodia depends on the focal adhesion signalling complexes formed following laminin/integrin binding [43] . Paxillin has a central role as a multi-domain scaffold protein, which promotes a complex interaction of signalling proteins and cascades. Downstream of the paxillin signalling complex is the dynamic subcellular regulation of Rac1-GTP levels. FRET analysis of Rac activity kinetics in SCs seeded on a laminin substrate and on axons identified an initial local Rac activation then suppression of Rac-GTP during elongation [44] . Rac-GTP dynamics and the resulting cytoskeletal reorganization are regulated in part by the Crk family of adaptor proteins that integrate signals from both adhesion proteins and growth factor receptors [45] . Paxillin mediates the activation of phospho(Y221)-CrkII upon cell adhesion [46] , and phospho(Y221)-CrkII has a central role in targeting Rac-GTP to the membrane, which is required for the activation of downstream Rac signalling pathways [47] . Phospho-Y118 Paxillin and Phospho(Y221)-CrkII levels in SCs, as well as Rac-GTP levels in SC-DRG cocultures, are significantly reduced by Lck inhibition ( Fig. 2 ). Finally, it has been suggested that cytoskeletal reorganization and radial lamellipodia formation in SCs requires an upregulation of active Rac1 (refs 19 , 21 ). However, the signalling pathway that mediates this ‘extra’ elevation in Rac1-GTP levels has not been elucidated so far. Here, we show that Lck is the molecular ‘switch’ that mediates signalling pathways, which include paxillin and CrkII, to elevate Rac1-GTP levels in response to β1-integrin signalling, leading to the formation of radial lamellipodia and the process of axonal sorting. As Lck signalling regulates cytoskeletal dynamics and migration of SCs, we hypothesized that inhibition of Lck would also affect the timing of SC myelination, which depends on the proper extension of cytoplasmic processes and membrane wrapping. Oct-6 expression is induced by axonal contact and is primarily expressed in late premyelinating and promyelinating SCs before the upregulation of Egr2 (ref. 48 ). In both myelinating DRG explants and P5 Lck −/− sciatic nerves, Oct-6 expression levels are decreased as compared with WT cultures and nerves, which may be the result of defects in axonal sorting and ensheathment of axons in Lck −/− SCs. In DRG explants, fewer SCs initiated the myelination programme ( Fig. 5 ) and in the Lck −/− mouse myelination is delayed, the myelin is thinner and there are defects in myelin architecture ( Figs 6 and 7 ). We propose that the delay in axonal sorting and extension due to lack of Lck signalling results in reduced expression of Oct-6 in Lck −/− SCs. This effect can be attributed directly to regulation of Oct-6 expression by Lck or indirectly because of the reduced rate of SC migration, which results in delayed initiation of the myelination-specific transcriptional programme. Our electron microscopy data confirm the delay in myelination in Lck −/− mice that correlates with the reduced expression of Oct-6 at the same time intervals. In addition, electron microscopy of the Lck −/− sciatic nerves reveals thinner myelin and numerous aberrant myelin outfoldings that are sustained in older animals, suggesting that Lck signalling may participate in myelin growth control in SCs. Myelin outfoldings have been found in many peripheral neuropathies including chronic inflammatory demyelinating neuropathy, different forms of Charcot-Marie-Tooth (CMT) and in paraproteinemic neuropathy [49] . This suggests that Lck may be part of a pathway that regulates the integrity of the myelin sheath in the PNS. In conclusion, we show that Lck has a crucial role in SC biology. It fine-tunes the cytoskeletal rearrangements of SCs through a paxillin-CrkII-Rac1 signalling pathway. Lck is the signalling ‘switch’ that upregulates Rac1 activity levels to induce formation of radial lamellipodia, which is a prerequisite for axonal sorting and myelination. Moreover, Lck signalling is required for the proper timing of myelination and the establishment of the correct thickness and integrity of the myelin sheath. Our data introduce Lck in the forefront of the signalling intermediates that regulate glial cell migration and cytoskeletal dynamics in the nervous system. Animal use and care C57/B6 WT mice and Lck −/− mice were obtained from Jackson Labs and maintained according to the NIH Guide for the Care and Use of Laboratory Animals. Lck −/− congenic mice were maintained on a C57/B6 background and all in vivo experiments used age-matched control animals. All animal use protocols were approved by the Institutional Animal Care and Use Committee of the Weis Center for Research, Geisinger Clinic. Primary cell culture treatments and transfections Isolation of rat DRG neurons, RSC cultures and myelination protocols were described earlier [50] , [51] . See Supplementary Methods for generation of mouse DRGs and SC cultures. Laminin activation of Lck was assessed by the addition of 15 μg ml −1 human placental laminin (Sigma) or mouse EHS laminin (Life Technologies) for 10 min or by seeding SCs on plates coated with 10 μg ml −1 laminin. For pharmacological inhibition of Lck, cultures were incubated with 500 nM Lck inhibitor (A770041, a generous gift from Abbott Biochemicals). This concentration does not inhibit Fyn, Lyn or Src tyrosine kinase [31] ( Supplementary Fig. S2 ). For overexpression studies, 1.5 × 10 6 RSCs were transfected with 300 nM siRNA pool ITGB1 (Dharmacon) with or without 2 μg mouse Lck complementary DNA (Origene) using nucleofection (Lonza). Cells were plated in SC media for 2 days then seeded on laminin-coated dishes (10 μg ml −1 ) for 3.5 h before lysis. For Lck siRNA interference studies, RSCs were transfected with Silencer Select scrambled CTL siRNA or rat Lck siRNA (Ambion) using Dharmafect reagent according to the manufacturer’s protocol (Dharmacon). Cells were cultured for 3 days then seeded on DRG cultures. BiFC analysis Fluorescent fusion proteins were produced using ITGB1 (GeneCopeia) and Lck (Origene) after amplification by PCR and subcloning into YFP(1-158)pcDNA1/Amp and YFP(159-238)pcDNA1/Amp (a generous gift from C. H. Berlot PhD) [27] . See Supplementary Methods for the detailed explanation of BiFC constructs. Both constructs were sequenced and protein expression was verified in Cos7 cells. Constructs were transfected into Cos7 using Fugene (Roche) and cells were imaged at 48 h post transfection. RSCs were transfected with Nucleofection (Lonza) and imaged after 48 h of protein expression. Intensity measurements of Cos7 expressing YFP constructs were measured from photomicrographs collected at a 3-s exposure with a gain of 1. The border of each cell was traced using ImageJ (NIH) and fluorescence intensity was calculated from the average pixel intensity of the entire cell. Instrument background was subtracted from each cell by subtracting the fluorescence intensity of a cell-free region multiplied by the area of the cell. Thirty-five cells from each coverslip were analysed from two independent experiments. As the expression of either YFP construct alone does not produce an active chromophore, this intensity level (<5) represents cell autofluorescence, and cells with average intensity levels below 5 were not included in the average fluorescence intensity calculation of the coexpression experiments. Live cell imaging RSCs were seeded on coverslips coated with 10 μg ml −1 laminin and imaged with on a Zeiss Axiovert microscope every 2 min for 2 h using Zeiss Axiovision software. Phase contrast images were compiled to mov movie files. For axonal migration studies, RSCs transfected with green fluorescent protein expression plasmid (Lonza) were seeded on DRG axons and allowed to attach for 2 h before the addition of treatments. Cultures were imaged every 10 min for 24 h and movies were made as above. Cell-spreading assay using electrical impedance The xCELLigence system (Roche) was used to monitor cell-electrode impedance during RSC treatment with Lck inhibitor. Electrical impedance due to cell spreading is presented as cell index. Cells were seeded on laminin-coated wells of the RTCA E-plate (xCELLigence Roche) and allowed to attach and spread to reach equilibrium. Treatment with DMSO (CTL), 200 and 500 nM Lck inhibitor were then added in the respective wells and the plate was returned to the analyser at 37 °C. Measurements were taken every 15 s for 2 h and every 1 min thereafter. Cell index data were normalized to the measurements just before adding treatment conditions and the average of four experiments was calculated. For the cell migration assays, equal amounts of cells were seeded in a RTCA CIM-16 plate (xCELLigence, Roche) in serum-free media allowed to attach for 1 h then returned to the analyser at 37 °C. As cells migrated to the lower chamber containing 10% serum media, measurements were taken each minute for 5 h. Cell index data was plotted over time and the slope between 2 and 4 h was calculated using RTCA DP software. Rac1-GTP pull-down assay DRG explants cultured on individual coverslips were seeded with 150,000 RSCs and treated continuously with DMSO alone or 500 nM Lck inhibitor for 3 days. Ten coverslips per condition were lysed and combined for each pull-down assay. Rac1-GTP pull-down was conducted according to the manufacturer’s directions (Millipore) and total lysates and pull-down samples were separated on a 4–12% SDS–polyacrylamide gel electrophoresis (SDS–PAGE) gel and immunoblotted for total Rac1 and actin. Immunoprecipitation and western blotting For immunoprecipitation studies, cultures were lysed in 1 × RIPA buffer containing phosphatase and protease inhibitors (Sigma). Lysates were cleared by centrifugation and precleared for non-specific binding by rotating with beads alone before primary antibodies against Lck (Millipore), Fyn, Lyn or Src (Cell Signaling) were added to the cleared lysates and rotated overnight at 4 °C. TrueBlot anti-rabbit IgG beads (eBioscience) or Protein G Dynabeads (Invitrogen) were added to the lysates and immunoprecipitates were washed then solubilized with 2 × SDS buffer, boiled and loaded on 8% SDS–PAGE gels and processed as described below. For total cell lysates, cultures were lysed in 1 × SDS lysis buffer containing phosphatase inhibitor and protease inihibitor (Sigma). Sciatic nerves were frozen in liquid nitrogen and homogenized in 1 × SDS lysis buffer. Lysates were cleared by centrifugation and the supernatants were collected and frozen at −80 °C. Samples were separated on 8% or 4–12% SDS–PAGE gels (NuPAGE), transferred onto nitrocellulose and immunoblotted. The following primary antibodies were used: phospho(Y418)-Src family, Lck(D88), Src, Fyn, Lyn, phospho(Y118)-paxillin, phospho-p44/42 MAPK (Cell Signaling Technology), β1-integrin and Lck(3A5 clone, Millipore), Egr2/Krox-20 (Covance), Oct-6 (Origene), glyceraldehyde 3-phosphate dehydrogenase (GAPDH; a kind gift of D Carey) and β-actin (Sigma). Secondary antibodies were horseradish peroxidase-conjugated goat anti-mouse and goat anti-rabbit (Cell Signaling) and donkey anti-goat (Jackson Immunolabs). Phospho(Y394)-Lck, a custom phospho-specific polyclonal antibody, was generated against the Lck active site and affinity-purified against non-phosphorylated Lck, and Fyn and Lyn active sites (Thermo-Fisher). Semi-quantitative analysis was conducted with FluorChem SP analytical software. Statistical significance was determined by two-tailed Student’s t -test. Representative full-length western blots are shown in the Supplementary Information ( Supplementary Fig. S6 ). Real-time qPCR Total RNA from SC-DRG myelinating cocultures treated with or without Lck inhibitor (three cultures per sample) was extracted using Trizol and treated with RNase-free DNAse I. cDNA was synthesized using the High Capacity RNA to cDNA kit (Applied Biosystems). Quantitative PCR was performed using Taqman Gene Expression Assays to assess message levels using verified Taqman probes for Oct-6, cJun, Egr2 and GAPDH (Applied Biosystems). No-template controls were also run and showed no contaminating DNA. Relative mRNA levels were normalized to GAPDH and two samples per group were quantified using the comparative C t method and fold change was calculated compared with WT samples. Immunocytochemistry Cells were fixed with 4% formaldehyde and permeabilized with 0.1% Triton-X100 or methanol. The following primary antibodies were used: MBP (Covance), neurofilament (Encor Biotechnology), ezrin, phospho(Y118)-paxillin (Cell Signaling) and Sox10 (R&D Systems). The cultures were then washed and incubated with AlexaFluor-488-conjugated goat anti-mouse IgG (Life Technologies), rhodamine-conjugated goat anti-chicken IgG (Jackson Immunochemicals) or AlexaFluor-576-conjugated goat anti-rabbit IgG (Life Technologies). Cultures were costained with 4′,6-diamidino-2-phenylindole. Images were captured with a Zeiss Axiovert inverted microscope equipped with Apotome and a high-resolution digital camera. For lamellipodia analysis, cultures were fixed with 4% formaldehyde and permeabilized with 0.1% Triton X-100, blocked with 1% bovine serum albumin in PBS and incubated with phalloidin-rhodamine (Life Technologies). Statistical analysis of myelination Photomicrographs were taken at × 10 magnification (10 fields per coverslip) and numbers of MBP+ segments were counted per coverslip. Internodes were measured using ImageJ software (NIH) and counted according to length. Standard deviation was calculated from seven cultures, and unpaired two-tailed Student’s t -test was performed. Electron microscopy and g-ratio analysis Isolated sciatic nerves were fixed by perfusion with 3% glutaraldehyde in phosphate buffer pH 7.4 at 4 °C. Nerves were then postfixed in 2% osmium tetroxide in 100 mM phosphate buffer, dehydrated in ethanol and embedded in Epox812 (Fullam, Latham, NY). For ultrastructural analysis, ultrathin section were cut, placed on copper grids, stained with lead citrate and uranyl magnesium acetate, and examined in Jeol (Peabody, MA) JEM-1200EX transmission/scanning electron microscope. To calculate g-ratios, we measured the ratio of the axonal diameter to the diameter of the myelinated fibre. We used EM photomicrographs from sciatic nerves of three WT and three Lck −/− mice for each time interval and measured ~1,000 axons from each group. The results are presented as average ±s.d. Semithin sections were cut and stained with toluidine blue and × 40 photomicrographs were taken. More than 1,000 axons per sciatic nerve cross-section were counted and the percentage of axons with aberrant myelin looping was calculated. Two animals for each time point were analysed. The results are presented as average ±s.d. How to cite this article: Ness, J. K. et al . Lck tyrosine kinase mediates β1-integrin signalling to regulate Schwann cell migration and myelination. Nat. Commun . 4:1912 doi:10.1038/ncomms2928 (2013).